Optically rewritable patterns of nuclear magnetization in gallium arsenide The control of nuclear spin polarization is important to the design of materials and algorithms for spin-based quantum computing and spintronics. Towards that end, it would be convenient to control the sign and magnitude of nuclear polarization as a function of position within the host lattice. Here we show that, by exploiting different mechanisms for electron–nuclear interaction in the optical pumping process, we are able to control and image the sign of the nuclear polarization as a function of distance from an irradiated GaAs surface. This control is achieved using a crafted combination of light helicity, intensity and wavelength, and is further tuned via use of NMR pulse sequences. These results demonstrate all-optical creation of micron scale, rewritable patterns of positive and negative nuclear polarization in a bulk semiconductor without the need for ferromagnets, lithographic patterning techniques, or quantum-confined structures. Control of electron spins in semiconductors impacts the design and analysis of both solid-state quantum computation schemes and spintronics devices [1] , [2] . In both applications, the electron spins are subject to internal magnetic fields that arise from nuclear spins. The small energy separation between nuclear spin states leads to a highly disordered, fluctuating spin ensemble that contributes significantly to electron spin decoherence, thereby limiting the fidelity of quantum computation. If the nuclear spins are polarized, their magnetic field acts on electron spins to produce an effective, static field in addition to the fluctuating component. Spatial control of this internal field is a prerequisite to coherent control of electron spin currents in spintronics devices [3] . Although patterns have been imprinted via ferromagnetic heterostructures [4] , [5] , and nanometer-scale control has been achieved by a variety of methods in quantum-confined semiconductors [6] , [7] , no general scheme for controlling internal nuclear fields has yet been developed for unstructured, bulk semiconductors. Optical excitation for the crafted preparation of nuclear polarization Ī z in semiconductors has a history extending back several decades [8] . Previous work focussed on the selection rules for excitation of spin-polarized electrons in GaAs, and the subsequent exchange of these electrons with spins bound at recombination centres [9] . These bound electrons have a strong contact hyperfine interaction with nearby nuclei that undergo dynamic nuclear polarization (DNP) driven by spin-exchange modulation of the hyperfine field. The DNP rate decays exponentially with distance from the recombination centre, and scales linearly with probability of trapping at a recombination centre [10] , [11] . Both the magnitude and sign of the polarization of nuclei undergoing DNP may be controlled by the polarization of the incident light. More recently, we identified a second mechanism [12] , [13] for nuclear polarization that arises from the interaction of a nuclear electric quadrupole moment with fluctuating electric field gradients at a recombination centre. These gradients arise from the spin-exchange process at recombination centres and result in a positive nuclear polarization by facilitating thermal relaxation. The charge carrier dynamics that drive both polarization processes depend on optical absorption rate, which is a function of optical absorption coefficient and light intensity. In the regime (near and above gap), where the optical penetration depth is smaller than the sample thickness, the electron generation rate is strongly dependent on depth in the sample. Because both illumination intensity and penetration depth (via different wavelengths) are variable across several orders of magnitude in typical laboratory settings, these parameters may be used to 'tune' the recombination centre dynamics and control the sign and magnitude of nuclear polarization. Here we harness this control to create micron-scale patterns of nuclear polarization as a function of position and isotope. These patterns are easily rewritable, depend only on simple parameters of optical excitation, and may be easily manipulated with NMR pulse sequences. Internal nuclear fields An intuitive way to view how nuclear polarizations produce effective static fields for spintronics applications begins with the Hamiltonian governing the behaviour of electron spins in a semiconductor: The first term of this Hamiltonian is associated with the static field and applied resonant pulses. The second term represents the contact hyperfine interaction with the many ( N ) nuclei enveloped by the single electron wavefunction. We can separate the applied magnetic field, B , into its static z -component (the Zeeman field denoted B 0 ), and its time-dependent component (RF or microwave pulses, arbitrarily chosen to be along the x axis). We can also separate the hyperfine interaction with nuclei into a static component (which has non-zero magnitude only in the z -direction) and a fluctuating component: Control of the average nuclear polarization, Ī z , effectively controls the Zeeman field as a function of position in space: with . It is this spatially dependent field that will enable spintronic and quantum computing device technologies and experimental control of is the necessary prerequisite. To understand how control of can be used to create patterns of nuclear magnetization, we examine the two distinct mechanisms of nuclear polarization. The hyperfine-induced nuclear polarization rate by the electron spin-exchange mechanism in the high-field limit is [13] where a 0 is the Bohr radius, Γ is the probability of a trapped electron at a recombination centre, r is the distance of a nucleus from the recombination centre, γ N is the nuclear gyromagnetic ratio, τ H is the correlation time for fluctuations of the hyperfine field, and ω H is the frequency associated with a nuclear-electron 'flip-flop' transition. In contrast, the quadrupolar polarization mechanism occurs due to modulation of the electric field gradients (EFGs) around recombination centres. These modulations are caused by the alternation between the ionized and neutral state of the recombination centre due to electron capture and recombination [13] . This modulation couples the nuclear Zeeman energy reservoir to the kinetic energy reservoir of the electrons, which rapidly equilibrates with lattice phonons [14] . Therefore, this mechanism always drives nuclei towards a positive spin temperature. The angular and radial dependence of the polarization rate are subtle, but in the high field limit the angular dependence of the total relaxation rate disappears and the rate is given by [13] where Q is the quadrupolar moment of the nucleus, R 14 is the electrostatic antishielding factor, ω N is the NMR frequency, and τ Q is the correlation time of fluctuations of the EFGs. The radial factor s ( r ) is given by . For this mechanism, the optimum recombination centre occupation probability is 50% and the rate decreases to zero as Γ approaches unity. Defining the ratio of the two relaxation timescales as and using [13] , we have (see equations (10), (11), (12), (13), (14) and (15)) From this relationship, we model the transport of nuclear spin polarization around a given recombination centre as where I Q ,0 is the equilibrium nuclear spin polarization via the quadrupolar mechanism and I H ,0 is the steady-state polarization due to the hyperfine mechanism (equations (17), (18) and (19)). Spin diffusion (characterized by the diffusion coefficient D ) is fast relative to the direct polarization rate outside the Bohr radius, where the magnitude of the electron wavefunction is negligible, so gradients of I z are neglected and the last term in equation (8) is zero. Integrating all terms in equation (8) over the sphere associated with a single recombination centre ( ) gives the polarization per recombination centre. As both polarization rates are very small as r approaches R , we approximate the limit of this integral as R →∞ . Equation (8) then yields the solution for polarization per unit volume. Stray-field imaging NMR imaging is a well-established technique that maps spatial information to the frequency domain by means of a magnetic field gradient. Nuclear spins at different positions within the inhomogeneous field may be identified by their different NMR frequencies. Here we employ a one-dimensional imaging technique known as stray-field imaging (STRAFI) [15] . The STRAFI experiment makes use of the large gradients available in the stray field of a superconducting NMR magnet. A schematic of the experimental set-up is shown in Fig. 1 . With a natural NMR linewidth of ~4 kHz for 69 Ga and a gradient of ~19 T m −1 , we achieved spatial resolution in the z -direction of 20 μm. As shown in the pulse diagram of Fig. 1 , data are acquired by first saturating the spin transitions with a series of RF pulses, after which the sample is illuminated with circularly polarized near-gap irradiation followed by signal acquisition via a π/2 pulse and inductive detection of the transverse magnetization. 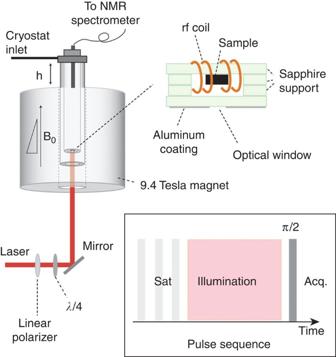Figure 1: Stray-field apparatus for imaging nuclear magnetism. The strong gradient in the stray field of a superconducting magnet provides the means for NMR imaging in one-dimension. Circularly polarized illumination is directed to the sample through an optical window on the sapphire sample support. Inset: the NMR pulse sequence including saturation, illumination and detection. Figure 1: Stray-field apparatus for imaging nuclear magnetism. The strong gradient in the stray field of a superconducting magnet provides the means for NMR imaging in one-dimension. Circularly polarized illumination is directed to the sample through an optical window on the sapphire sample support. Inset: the NMR pulse sequence including saturation, illumination and detection. Full size image The STRAFI data in Fig. 2 correspond directly to the sign and magnitude of nuclear magnetization as a function of depth in the sample. At the lowest illumination intensity (4 mW cm −2 ), the polarization is positive throughout the sample, and is nearly independent of helicity, consistent with the bulk experiments reported previously [12] . At the highest illumination intensity (102 mW cm −2 ) the sign of the polarization throughout much of the sample may be controlled with light polarization, consistent with many previous bulk studies in this regime [8] , [16] . Here the intermediate regime is of interest. In this regime of intermediate illumination intensity, using σ + polarization, regions of opposite spin polarization are created within close proximity in the GaAs wafer. Neglecting for now the positive signals immediately at the illuminated surface (discussed later) a negative signal is found close to the surface of the sample where absorption is greatest and electron spin exchange dominates the nuclear polarization process. A positive signal emanates from that portion of the wafer where the light intensity has decayed. In these regions of reduced absorption, the recombination centre occupation fraction decreases such that the quadrupolar polarization mechanism is dominant. By adjusting the wavelength of light ( Fig. 3 ), we vary the optical penetration depth, controlling the length scale of the patterns of polarization. For example, using 810 nm irradiation, our analysis reveals that we created features ~40 μm wide. 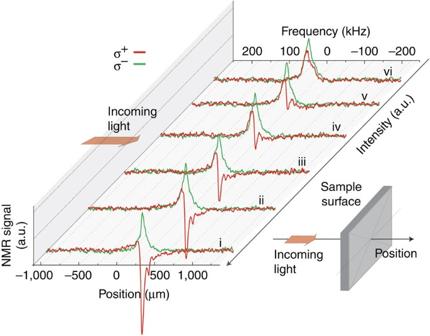Figure 2: Spatial patterns of69Ga nuclear magnetism as a function of laser intensity. NMR images of69Ga nuclear polarization at (i) 102 mW cm−2, (ii) 51 mW cm−2, (iii) 37 mW cm−2, (iv) 29 mW cm−2, (v) 12 mW cm−2and (vi) 4 mW cm−2. Red curves correspond toσ+ helicity, green curves correspond toσ−and the wavelength is 825 nm. The origin is chosen to approximately coincide with the semiconductor wafer surface. Inset: incoming light illuminates the sample from the left (coincident with higher frequencies in our set-up, see upper horizontal axis). Figure 2: Spatial patterns of 69 Ga nuclear magnetism as a function of laser intensity. NMR images of 69 Ga nuclear polarization at (i) 102 mW cm −2 , (ii) 51 mW cm −2 , (iii) 37 mW cm −2 , (iv) 29 mW cm −2 , (v) 12 mW cm −2 and (vi) 4 mW cm −2 . Red curves correspond to σ + helicity, green curves correspond to σ −and the wavelength is 825 nm. The origin is chosen to approximately coincide with the semiconductor wafer surface. Inset: incoming light illuminates the sample from the left (coincident with higher frequencies in our set-up, see upper horizontal axis). 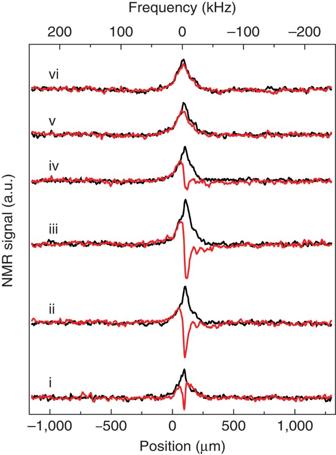Figure 3: Controlling the length scale of nuclear magnetism with illumination wavelength. Stray field images of nuclear polarization for69Ga as a function of irradiation wavelength for an illumination intensity of 37 mW cm−2after 10 min. (i) 810 nm, (ii) 820 nm, (iii) 825 nm, (iv) 830 nm, (v) 835 nm, (vi) 855 nm. Red curves correspond toσ+ helicity and black curves correspond toσ−. Decreasing the wavelength to 810 nm (i) provides the shortest length scale for polarization patterning. Our analysis indicates that the width of the negative polarization region associated with this spectrum is ~40 μm. Full size image Figure 3: Controlling the length scale of nuclear magnetism with illumination wavelength. Stray field images of nuclear polarization for 69 Ga as a function of irradiation wavelength for an illumination intensity of 37 mW cm −2 after 10 min. (i) 810 nm, (ii) 820 nm, (iii) 825 nm, (iv) 830 nm, (v) 835 nm, (vi) 855 nm. Red curves correspond to σ + helicity and black curves correspond to σ −. Decreasing the wavelength to 810 nm (i) provides the shortest length scale for polarization patterning. Our analysis indicates that the width of the negative polarization region associated with this spectrum is ~40 μm. Full size image Modelling Without detailed knowledge of the electron recombination dynamics, optical absorption at high-field and low temperature, and kinetics of electron capture at recombination centres, it is difficult to quantitatively model the dependence of the patterns on illumination wavelength and intensity. However, assuming a single binary recombination mechanism and Langmurian binding of free electrons to recombination centres, combined with literature values for optical absorption [10] , we reproduce the shape of the STRAFI images as a function of illumination intensity for a given wavelength ( Fig. 4 ). We also note that, for most experimental conditions, there is a region of positive polarization localized at the irradiated surface. We attribute this to a depletion layer of low recombination centre occupation near the surface where the quadrupolar mechanism dominates. Briefly, defect states pin the Fermi-level mid gap at the surface and an electric field extends from the surface into the bulk. Recombination centres may be ionized in the regions where the electric field exceeds ~5,000 V cm −1 (ref. 17 ). The approximate width of the depletion layer is given by (ref. 14 ) where ε is the dielectric constant, ε 0 is the vacuum permittivity, φ 0 is the potential of the pinned Fermi-level at the surface, and ρ is the charge carrier density. To theoretically reproduce STRAFI images, a depletion layer of 50 μm was included in the simulations. Assuming the Fermi-level is pinned mid-gap, this corresponds to a carrier concentration of ~10 14 cm −3 , which is similar to the free electron concentrations predicted by the simplified model for a semi-insulating sample at low temperature with optical illumination. Given this very simplistic model, the agreement with experiment ( Fig. 3 ) is nearly quantitative. 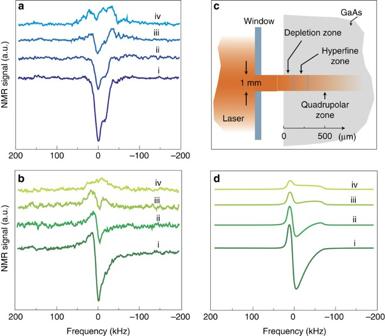Figure 4: Understanding the roles of quadrupolar and hyperfine polarization. Stray field images of nuclear polarization for (a)71Ga and (b)69Ga.69Ga, the isotope with the larger quadrupolar moment and smaller magnetic moment, transitions from the (negative) hyperfine regime to the (positive) quadrupolar regime at higher irradiation intensity. (c) Spatial patterns are due to the various 'zones' where either the hyperfine or quadrupolar mechanism may dominate. (d) Simulated STRAFI images for69Ga capture the changing shape of the distribution of nuclear polarization with illumination intensity. For (a), the intensities are (i) 75 mW cm−2, (ii) 35 mW cm−2, (iii) 10 mW cm−2, (iv) 5 mW cm−2. For both (b) and (d) the intensities are (i) 83 mW cm−2, (ii) 38 mW cm−2, (iii) 14 mW cm−2, (iv) 6 mW cm−2. Figure 4: Understanding the roles of quadrupolar and hyperfine polarization. Stray field images of nuclear polarization for ( a ) 71 Ga and ( b ) 69 Ga. 69 Ga, the isotope with the larger quadrupolar moment and smaller magnetic moment, transitions from the (negative) hyperfine regime to the (positive) quadrupolar regime at higher irradiation intensity. ( c ) Spatial patterns are due to the various 'zones' where either the hyperfine or quadrupolar mechanism may dominate. ( d ) Simulated STRAFI images for 69 Ga capture the changing shape of the distribution of nuclear polarization with illumination intensity. For ( a ), the intensities are (i) 75 mW cm −2 , (ii) 35 mW cm −2 , (iii) 10 mW cm −2 , (iv) 5 mW cm −2 . For both ( b ) and ( d ) the intensities are (i) 83 mW cm −2 , (ii) 38 mW cm −2 , (iii) 14 mW cm −2 , (iv) 6 mW cm −2 . Full size image Engineered nuclear magnetization We investigated the isotope dependence of the patterning process ( Fig. 4a,b ). As expected, the isotope with the larger quadrupole moment and smaller gyromagnetic ratio required greater irradiation intensity to transition from positive to negative polarization. Comparing the intermediate irradiation intensity data in Fig. 4a,b (for example 14 mW cm −2 ), we observed the unique situation where different isotopes of the same chemical species have opposite polarization at the same location in the sample, suggesting the ability to create heteronuclear spin order via dipolar or indirect J-coupling [18] . Furthermore, optical pumping can be combined with NMR pulse sequences to further control nuclear polarization. As a proof of principle, we combined periods of optical pumping of varied intensity and wavelength with NMR π pulses to isolate regions of hyperfine- and quadrupolar-induced polarization ( Fig. 5 ). Many sophisticated NMR pulse sequences exist that interconvert various types of spin order and coherence, which may be combined with wavelength, intensity and helicity control of spatially patterned polarization to create a range of spatially dependent spin dynamics. 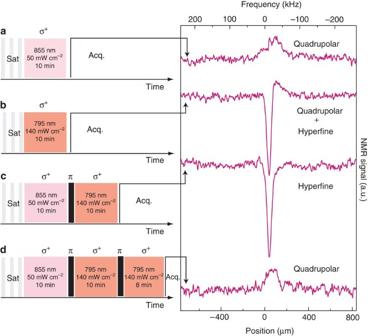Figure 5: Engineering nuclear magnetism. Optical pumping parameters may be chosen so that (a) quadrupolar relaxation dominates, or (b) both mechanisms act simultaneously on different regions in the sample. By combining periods of optical pumping with different intensity and wavelength, separated byπpulses, only the (c) hyperfine or (d) quadrupolar polarized regions remain. All images correspond to69Ga polarization. Figure 5: Engineering nuclear magnetism. Optical pumping parameters may be chosen so that ( a ) quadrupolar relaxation dominates, or ( b ) both mechanisms act simultaneously on different regions in the sample. By combining periods of optical pumping with different intensity and wavelength, separated by π pulses, only the ( c ) hyperfine or ( d ) quadrupolar polarized regions remain. All images correspond to 69 Ga polarization. Full size image We have demonstrated an all-optical method to create patterns of polarized nuclear spins from millimeter to micron length scales. All regimes are easily accessible under typical laboratory conditions. Rastering of the laser beam will provide an additional two dimensions of spatial control, and combining NMR pulse sequences with optical irradiation gives a general scheme for creating patterns. These patterns persist for a timescale equal to the nuclear spin-lattice relaxation time, minutes to hours under these conditions, which is more than sufficient for any NMR pulse sequence or quantum computing protocol. Patterns may be erased (saturation), reoriented (θ° RF pulses), or converted to various types of spin-order through available NMR pulse sequences. We also note that for applications where the surface depletion layer is undesired, Fermi-level pinning does not occur, for example, on a freshly cleaved (110) GaAs surface [14] and may be avoided with an inert atmosphere or protective encapsulation. We call specific attention to the possibility of using patterned nuclear polarization to create effective Zeeman fields in electron-spin based devices. Such fields may be used to selectively tune the resonance frequency of confined electrons. Coherent electron spin rotations have already been achieved [2] , by causing electrons to drift through a region of magnetized nuclei. Micron-level, three-dimensional patterning of nuclear magnetism gives a new degree of freedom in semiconductor spintronics that will be easily integrated into existing device architectures with optical and electrical control. We also note that the relative rates of the two polarization mechanisms are a function of distance from a given recombination centre. This suggests the possibility of achieving patterned polarization on a length scale similar to the Bohr radius (~10 nm in GaAs). For an s -orbital hydrogenic wavefunction, the hyperfine polarization rate is greatest where the electron density is highest (near the recombination centre) and becomes small outside the Bohr radius. In contrast, the quadrupolar mechanism relies on fluctuations in the gradient of the electric field. Symmetry considerations dictate that no gradients exist at the centre of a spherically symmetric environment, so the behaviour near the recombination centre is dominated by the hyperfine interaction. The quadrupolar interaction reaches a maximum on the order of the Bohr radius from the defect site and decays less rapidly as a function of distance. Future studies will investigate the local distribution of nuclear polarization near defects. Stray-field NMR imaging NMR images for 71 Ga and 69 Ga are obtained using the stray field of a 9.4 T superconducting NMR magnet. The RF pulse sequence is SAT- τ L – π /2, where SAT is the saturation of the spin transitions by a series of pulses, τ L is the irradiation time, and the final π /2-pulse (8 μs) converts the nuclear polarization into observable coherences. The sample is a (100) wafer of semi-insulating GaAs (American Crystal Technologies) with resistivity greater than 10 7 Ωcm. To ensure good thermal conductivity, we use Apiezon N grease to mount the sample of thickness 350 μm atop a long, rectangular sapphire strip. The strip bridges the opposite sides of an ~3 cm diameter opening at the centre of a thin copper plate, whose orientation relative to the static magnetic field can be (slightly) adjusted using screws connected to the outside of the cryostat via long G10 rods. A split-coil surrounding the sample (and sapphire wafer) as part of a purpose-made cryogenic probe serves as the radio-frequency source. The coil shape and size are chosen so as to optimize the sample filling-factor while avoiding making physical contact with the support wafer or GaAs crystal. As shown in Fig. 1 , the area illuminated by the laser beam on the sample surface is defined by a proximal 1×1 mm 2 square window etched on an aluminum-coated sapphire strip aligned to coincide with the coil central gap. We use an optical expander to widen the laser beam so as to reach a 5-mm-diameter waist before the Al window, thus ensuring homogeneous intensity over the optically pumped surface. We control the beam helicity using a linear polarizer and a quarter wave plate. We illuminate the sample at 6.5 K through the quartz windows at the bottom of a modified Janis–Varitran cryostat, and use the G10 rods protruding at the upper end of our NMR probe to align the GaAs wafer, perpendicular to the direction of the static magnetic field. To accomplish this, we adjust the copper plate orientation while monitoring the part of the laser beam reflected from the aluminum-coated sapphire; this method allows us to reach a sample orientation precision better than half a degree. In preparation for the optical-pumping experiments reported herein, we conducted extensive preliminary experiments aimed at determining the magnetic field gradient as a function of the sample position within the magnet bore. For this purpose, we recorded the 71 Ga NMR signal from a 350-μm-thick GaAs wafer at room temperature for multiple displacements of the cryostat from its rest position atop the magnet. NMR spectra were attained using a simple excitation–acquisition protocol with 1-μs-long RF pulses so as to ensure the broadest excitation bandwidth possible. The magnetic field gradient is linear over the sample volume and exceeds 70 T m −1 at the maximum displacements we tested. For the present optical pumping experiments, we use a somewhat moderate gradient (~19 T m −1 ) as a reasonable tradeoff between spatial resolution and signal-to-noise ratio for typical illumination times (~10 min). Unless otherwise noted, the illumination wavelength is 825 nm. Calculation of the polarization rate ratio The ratio between the rates of the hyperfine and quadrupolar polarization mechanisms around a given defect is labelled ' f ': In the high magnetic-field limit (ω H τ H ≫ 1), the hyperfine polarization rate is given by The quadrupolar polarization rate is which in the high magnetic field limit ( ω N τ Q ≫ 1) reduces to with Here ω N is the frequency associated with a Δ I z =1 nuclear spin transition and ω 2 ~2 ω N is the frequency associated with a Δ I z =2 transition. Using the high magnetic field limit for both polarization mechanisms, the ratio becomes Equilibrium and steady-state polarizations The quadrupolar polarization mechanism is driven by electron capture and recombination at recombination centres, thereby coupling the nuclear Zeeman energy reservoir to the electron kinetic energy reservoir. The electrons are assumed to thermalize rapidly, so that the electron kinetic temperature is equal to the lattice temperature. For a spin −3/2 system, the polarization is given by At 6 K for 71 Ga in a field of 9.4 T, this corresponds to a polarization of ~0.1% or a nuclear field of ~56 Gauss (ref. 5 ). The steady-state value for a spin-3/2 nucleus undergoing DNP induced by a contact hyperfine interaction is where Δ S z is the departure of S z from its thermal equilibrium value. This parameter is given by where S 0 is the polarization of electrons due to excitation selection rules, S eq is the thermal equilibrium polarization of electrons, and τ and T le , respectively, denote the electron recombination lifetime and spin-lattice relaxation time of electrons. Hyperfine-induced nuclear polarization in semiconductors has been measured to be of the order of 10% (ref. 19 ). 10% polarization in GaAs corresponds to a nuclear field of ~5,600 Gauss (ref. 5 ). How to cite this article: King, J. P. et al . Optically rewritable patterns of nuclear magnetization in gallium arsenide. Nat. Commun. 3:918 doi: 10.1038/ncomms1918 (2012).